Advantage of rare infanticide strategies in an invasion experiment of behavioural polymorphism Killing conspecific infants (infanticide) is among the most puzzling phenomena in nature. Stable polymorphism in such behaviour could be maintained by negative frequency-dependent selection (benefit of rare types). However, it is currently unknown whether there is genetic polymorphism in infanticidal behaviour or whether infanticide may have any fitness advantages when rare. Here we show genetic polymorphism in non-parental infanticide. Our novel invasion experiment confirms negative frequency-dependent selection in wild bank vole populations, where resource benefits allow an infanticidal strategy to invade a population of non-infanticidal individuals. The results show that infanticidal behaviour is highly heritable with genetic correlation across the sexes. Thus, a positive correlative response in male behaviour is expected when selection operates on females only and vice versa . Our results, on one hand, demonstrate potential benefits of infanticide, and on the other, they open a new perspective of correlative evolution of infanticide in females and males. Infant death at the hand of parents or other adults is a common phenomenon in many vertebrates [1] . The evolutionary basis of infanticidal behaviour has received a vast amount of interest both in evolutionary and behavioural ecology [2] , [3] , [4] , [5] , [6] . Many reasons have been suggested to explain this behaviour, which may differ between species and even between the sexes within a species. Furthermore, the function of killing offspring depends on whether an individual kills its own offspring or offspring of unrelated conspecifics [7] . Here we focus on the origin and maintenance of the latter case, that is, non-parental infanticide. At least three main hypotheses have been presented to explain the function of non-parental infanticide: resource competition, predation and sexual selection hypotheses [1] , [8] . According to the resource competition hypothesis infanticidal individuals or their kin may receive greater access to resources, such as food or a nesting site, if they kill the offspring of competitive breeders, whereas the predation hypothesis suggests offspring are simply killed for food. These two hypotheses are not mutually exclusive as eating infants could still be beneficial even if they were originally killed for another reason. The third hypothesis of sexual selection explains only male infanticide. It suggests that males kill the infants of other males in order to gain a reproductive advantage over their male rivals and reduce the time until a female next ovulates. In many rodent populations [1] including our study species, the bank vole ( Myodes glareolus ) [9] , a clear polymorphism in infanticidal behaviour exists; some individuals seem to be non-infanticidal, whereas others frequently kill the pups of conspecifics. One of the most promising evolutionary mechanisms that maintains this behavioural polymorphism is negative frequency-dependent selection, where rare types are favoured by selection [10] , [11] , [12] , [13] , [14] . An infanticidal polymorphism could thus arise when rare infanticidal or non-infanticidal invaders have invaded each other's populations [15] ( Fig. 1 ). Further, this idea is based on the assumption that the behavioural polymorphism (here infanticidal behaviour) is genetically determined. This assumption was tested here by the analyses of quantitative genetics. 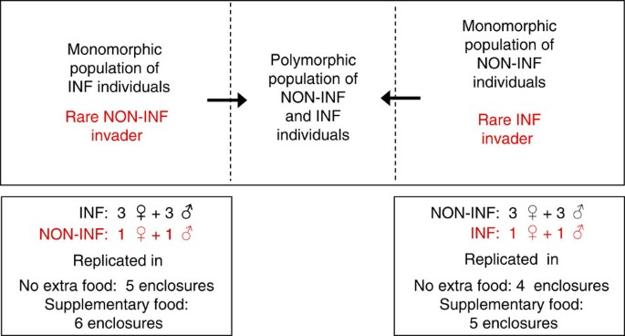Figure 1: The design of the invasion experiment. Negative frequency-dependent selection promotes polymorphism when rare mutants successfully invade monomorphic resident populations. In the factorial design of our invasion experiments, both infanticidal (INF) and non-infanticidal (NON-INF) individuals represented either resident or invader strategies, and the set up was replicated in enclosures with or without supplemental food supplies. Figure 1: The design of the invasion experiment. Negative frequency-dependent selection promotes polymorphism when rare mutants successfully invade monomorphic resident populations. In the factorial design of our invasion experiments, both infanticidal (INF) and non-infanticidal (NON-INF) individuals represented either resident or invader strategies, and the set up was replicated in enclosures with or without supplemental food supplies. Full size image Here we applied a novel experimental design ( Fig. 1 ) to test the hypothesis that negative frequency-dependent selection, coupled with the availability of food resources, determines the relative success of infanticidal tactics in field populations. This invasion experiment effectively tests whether a different infanticidal tactic can invade populations under different resource environments. Two factors in the experiment, the frequency of infanticidal tactics and food resources, were manipulated in 20 large outdoor enclosures. In 11 enclosures extra food was provided ad libitum and in 9 enclosures no supplemental food was provided. Furthermore, in each enclosure population the infanticidal tactics (infanticidal or non-infanticidal) were either rare (25%) or common (75%). We analysed the difference in infanticidal frequencies after selection between the founder population and their descendants. The analyses of quantitative genetics confirm a genetic polymorphism in infanticidal behaviour and, furthermore, the invasion experiment demonstrates negative frequency-dependent selection on infanticidal behaviour in wild populations of bank voles. We have showed that a rare infanticide type can invade a non-infanticidal population especially when food resources are limited. This supports model predictions [15] that resource benefits allow an infanticidal strategy to invade a population of non-infanticidal individuals. Genetic polymorphism Quantitative genetic analyses based on the infanticidal behaviour of parents (845 mothers and 772 fathers) and their offspring (481 females and 486 males) indicated high repeatability ( r =0. 77) of infanticidal behaviour and high additive genetic variance in infanticidal behaviour in our population of bank voles ( Table 1 ). The overall frequency of infanticide in the population was 61%, being slightly higher among females 66% than males 54% ( χ 2 =14.5, P <0.001). An average of the two sexes revealed a high heritability estimate for liability to infanticidal behaviour ( h 2 =0.71). The estimate of genetic correlation across the sexes was also relatively large ( r FM =0.62), which predicts a positive correlative response in the other sex even when natural selection only operates on the opposite sex. Table 1 Incidences of infanticidal behaviour among female and male offpring by male and female propositi in a laboratory population. 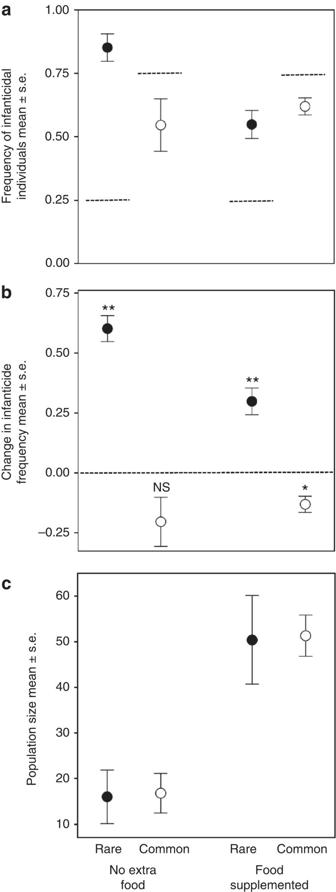Figure 2: Frequencies and numbers of infanticidal bank voles during the invasion experiment. (a) Frequency of infanticidal individuals in populations at the end of the breeding season. Closed circles show the mean number of voles in populations where infanticidal individuals were initially rare (and non-infanticidal individuals common); and open circles indicate the populations where infanticidal individuals were initially common (and non-infanticidal individuals rare) in founder populations. Dashed lines show the initial frequency of infanticidal tactics in each treatment. (b) Frequency change in infanticidal tactics with different food manipulations (for statistics seeTable 2). Asterisks indicate a significant difference (**P<0.01, *P<0.05) from the zero line. Infanticidal individuals can invade both food treatments when they are initially rare (closed circles;t=11.14,df=3,P=0.002;t=5.41,df=4,P=0.006; respectively), but more easily invade populations when food is limited (comparison between the food treatments:t=3.86,df=7,P=0.006). Instead, the rare non-infanticidal tactic (open circles) was significantly favoured only in the populations with supplemented food (t=5.41,df=4,P=0.012). (c) Population size increased with supplemental food (F=28.35,P<0.001), but was not affected by the initial frequency of infanticidal individuals in the population (F=0.018,P=0.895). NS, not significant. Full size table Negative frequency-dependent selection Frequency changes along the reproductive season in experimental populations indicate a clear benefit of rare invaders ( Table 2 ). In addition, there was also a significant interaction between initial frequency of infanticidal individuals and food availability. Consequently, it is easier for the infanticidal type to invade a population of non-infanticidal individuals when food resources are limited, and vice versa when food is abundant ( Fig. 2a,b ; Table 2 ). Overall, the initial frequency of infanticidal tactics in the founder populations did not affect population growth ( Fig. 2c ), only the proportion of individuals expressing the rare tactic increased significantly in both food treatments. This result may partly indicate an effective nest defence behaviour among infanticidal mothers, otherwise the number of recruits should decrease simultaneously with an increasing frequency of infanticidal individuals in the population [9] . Table 2 General linear model analysis of change in infanticidal frequency. Full size table Figure 2: Frequencies and numbers of infanticidal bank voles during the invasion experiment. ( a ) Frequency of infanticidal individuals in populations at the end of the breeding season. Closed circles show the mean number of voles in populations where infanticidal individuals were initially rare (and non-infanticidal individuals common); and open circles indicate the populations where infanticidal individuals were initially common (and non-infanticidal individuals rare) in founder populations. Dashed lines show the initial frequency of infanticidal tactics in each treatment. ( b ) Frequency change in infanticidal tactics with different food manipulations (for statistics see Table 2 ). Asterisks indicate a significant difference (** P <0.01, * P <0.05) from the zero line. Infanticidal individuals can invade both food treatments when they are initially rare (closed circles; t =11.14, df =3, P =0.002; t =5.41, df =4, P =0.006; respectively), but more easily invade populations when food is limited (comparison between the food treatments: t =3.86, df =7, P =0.006). Instead, the rare non-infanticidal tactic (open circles) was significantly favoured only in the populations with supplemented food ( t =5.41, df =4, P =0.012). ( c ) Population size increased with supplemental food ( F =28.35, P <0.001), but was not affected by the initial frequency of infanticidal individuals in the population ( F =0.018, P =0.895). NS, not significant. Full size image Both sexes responded equally to our resource manipulations ( Table 3 ; no significant interaction between sex, frequency and food) and frequencies of infanticidal females and males correlated positively in the populations ( r =0.686, N =19, P =0.001). Because of the positive genetic correlation between the sexes, selection for female infanticidal behaviour should result in the same response in males and vice versa . To date there is only weak evidence for the benefits of male infanticide and only relation to increased access to mates in natural populations of small mammals [1] . For example, killing pups does not shorten the time that females would re-enter oestrus in small mammals, as females are normally already pregnant when nursing their present pups. However, delayed implantation occurs in many rodents when rearing offspring [16] , therefore, by killing present unrelated pups soon after copulation, males may speed up the implantation of their own fertilized eggs. There are also some other benefits (for example, induced pregnancy block), which could be strong enough to maintain male infanticide in rodents [17] . Furthermore, the present results show that infanticide in male rodents can be partly a by-product of selection for female infanticide. Table 3 General linear mixed model analysis of the infanticidal status of individuals after the field experiment. Full size table In conclusion, the present results clearly support the hypothesis that competition for food resources can have a central role in the evolution of infanticidal behaviour. As reproductive success is constrained by food resources in many infanticidal species, including the bank vole [18] , infanticidal females should be able to increase their breeding success by killing the pups of competitors. However, infanticidal behaviour should also carry some other fitness costs and we find that non-infanticidal individuals can more effectively invade a population if food resources are not limited. Although the exact behavioural and physiological mechanisms are still unclear, we can conclude that the invasion success of different infanticidal tactics can vary according the level of food resources as well as the frequency of the opposite tactic in the populations. Study species The study species, the bank vole ( Myodes [Clethrionomys] glareolus ), is a small rodent species common in the northern Europe [19] . They mainly inhabit forests and fields feeding on forbs, shoots, seeds, berries, fungi and insects [20] . The density of breeding females is limited through their territoriality [21] , and at high densities, the maturation of young females is suppressed by social interactions among females [22] , [23] , [24] . In our study area, bank vole females give birth to a maximum of four litters during the breeding season, which lasts from late April to September. Litter sizes range from two to ten offspring [25] . Nursing lasts around 20 days after which the pups reach total independence from their mother. Females breed in postpartum oestrus, that is, they can become pregnant within a few hours after parturition. Thus, for individual females reproductive events such as parturition can occur at regular intervals throughout the breeding season. Bank vole males do not rear their offspring and male quality does not affect the amount of maternal care [26] ; hence, we can assume that genetic analyses are not biased by covariances between non-genetic maternal effects and genetic paternal effects. The patterns and amplitude of density variation show considerable geographical variability and both stable and cyclic populations are found in the bank vole [27] , [28] . The frequency of infanticidal tactics may differ according to population density or spatial and temporal variation in food resources, but to the best of our knowledge, the effects of these factors have not been reliably tested in the bank vole or other rodents. Individual infanticidal status The infanticidal behaviour of all bank vole individuals (second generation laboratory stock from wild ancestors) was tested in the Experimental Animal Unit of the University of Jyväskylä using the neutral arena procedure [29] . A newborn pup was placed in the middle of a standard mouse cage (43×26×15 cm 3 ) with a thin layer of clean sawdust and an adult test individual was introduced into the cage and placed under continuous observation. If the adult aggressively attacked the pup during the 30 min observation time it was considered infanticidal. Usually infanticidal individuals indicated clear aggression against the pup within 10 min, whereas non-infanticidal individuals typically inspected the pup several times during the test but did not harm it. If aggression against the test pup was expressed, the pup was immediately removed from the test arena and humanely killed. High repeatability ( F ratio, r =0.77) of infanticidal behaviour was confirmed by testing 44 individuals twice during a 1-month interval. Analyses of quantitative genetics In the analysis of quantitative genetics, we used the infanticidal status of 967 individuals (481 females and 486 males) and their mothers ( n =845) and fathers ( n =772). We analysed the effects of parental phenotypes on offspring phenotype by subjecting the infanticidal data to a logit analysis [30] ( Table 4 ). In this analysis, the existence of offspring infanticide was regarded as a response variable and father and mother phenotype as explanatory variables. Because the incidence of infanticide was slightly different for females and males, and because infanticidal behaviour of mothers and fathers seemed to be independent (contingency coefficient between sexes: C =0.072; P >0.05), we conducted separate analyses for the different sexes. The GLIM statistical package [31] was used to fit and determine the parameters of the logit models. We also estimated Akaike's information criterion (AIC) for each logit model to select the model with the highest information content. For logit models, this means choosing a model that minimizes AIC: where G 2 (X) is the likelihood ratio test statistic for testing the X model against the saturated model, r is the number of degrees of freedom for the X model and q is the degrees of freedom for the saturated model. Because q does not depend on the model, we used a slight modification of AIC : where [ q–r ] is the test degrees of freedom [30] . Minimizing AIC–q is equivalent to minimizing AIC . Table 4 Logit main factor models of parental phenotypes influencing offspring infanticidal behaviour in the laboratory. Full size table We assumed that infanticide is a polygenically and environmentally determined character and applied the 'threshold' model (for example, refs 32 , 33 , 34 ) to estimate the genetic parameters for it. The threshold model posits that the determination of the discontinuous variation in a character is a consequence of some underlying character, called the liability, which is itself continuously distributed. The model proposes that at some point along the liability distribution of a continuous trait, a threshold exists past which an individual shows the phenotypic character. Genetic parameters of liability could be estimated using data on the incidence of a character among relatives of infected individuals (known as propositi) and the incidence among relatives of controls. We estimated the parent–offspring regression for the liability of infanticide using the equation derived from ref. 35 : where i is the mean deviation of affected individuals from the population mean, and X and X R are the normal deviates of population and offspring of the threshold from the mean. Regression was estimated for each of four combinations: mother and female ( t FF ) and male offspring ( t FM ), and also for father and female ( t MF ) and male offspring ( t MM ). The heritabilities of liability may be computed as t/r , where r is the intraclass correlation (equivalent to the coefficient of relationship among relatives). Consequently, the heritability for females ( h 2 F ) was estimated as 2 t FF and for males ( h 2 M ) as 2 t MM . The corresponding values across sexes (2 t FM and 2 t MF ) include also genetic covariances between the opposite sexes [34] . The genetic correlation across the sexes was estimated as (Lynch and Walsh [34] ; p. 740): Field experiment The experiment was carried out at Konnevesi, central Finland (62°37′N, 26°20′E) in 20 outdoor enclosures (0.2 ha each; for details on the vegetation and construction of enclosures, see ref. 36 ). Each enclosure population was founded by eight voles (four females and four males) at the beginning of the breeding season (early June). In the experiment, two factors (the frequency of infanticidal tactics and food resources) were manipulated. In 11 enclosures extra food (sunflower seeds) was provided ad libitum at each trapping station (20 per enclosure) and in 9 enclosures no supplemental food was provided. Furthermore, in each enclosure infanticidal tactics were either rare or common ( Fig. 1 ). Frequency manipulations (rare: 25% and common: 75%) were constrained by breeding densities in the enclosures. The infanticidal status of founder individuals was tested using the behavioural trials described above. To increase the probability of discovering a genetic basis for the chosen tactics, only the individuals whose infanticidal tactic resembled that of both parents were selected for the experiment. However, we were unable to test how the laboratory measurement of infanticidal behaviour predicts infanticidal behaviour in the enclosures. All founder individuals were divided between the treatment groups randomly, for example, individual size did not differ between treatments at the beginning of the experiment (body mass: frequency P =0.265, food P =0.517; head width: frequency P =0.445, food P =0.860). After the breeding season (in September) all individuals were live-trapped and returned to the laboratory, where they were weighed to the nearest 0.1 g on a digital scale and head width was measured to the nearest 0.1 mm with a digital calliper. All recruits (708 offspring) were maintained in the laboratory for a month before infanticidal status was tested (see Methods above). During this habituation period food was provided ad libitum to diminish the direct effects of food manipulations on infanticidal status. We were able to test the infanticidal status of 278 female and 303 male offsprings, an average of 84% (range 69–100%) of the individuals from each enclosure. The proportion of tested individuals did not differ between the enclosures or the treatments (linear mixed model, P >0.05 for each). In the main statistical analyses ( Table 2 ), the change in infanticide frequency in each population during the experiment was explained by the initial frequency of infanticidal behaviour (rare or common) and food manipulation (supplemental food or no extra food) and their interaction. Ethical note The experiments were conducted with the permission of the Ethical Committee of Scientific Animal Experiments and the Provincial Administrative Board of Western Finland. The evaluation of the Ethical Committee was based on similar guidelines presented by The Association for Study of Animal Behaviour 32. The main criteria for the permit were to keep the number of tested animals and the severity of treatment, for each individual, as low as possible (see above). How to cite this article: Mappes, T. et al . Advantage of rare infanticide strategies in an invasion experiment of behavioural polymorphism. Nat. Commun. 3:611 doi: 10.1038/ncomms1613 (2012).